Direct visualization of a guest-triggered crystal deformation based on a flexible ultramicroporous framework Host–guest composites may exhibit abnormal and/or controllable physical properties that are unavailable for traditional solids. However, it is still very difficult to control or visualize the occupancy and motion of the guest. Here we report a flexible ultramicroporous coordination polymer showing exceptional guest-responsive thermal-expansion properties. The vacant crystal exhibits constant and huge thermal expansion over a wide temperature range not only in vacuum but also in air, as its ultramicroporous channel excludes air adsorption even at 77 K. More interestingly, as demonstrated by single-crystal X-ray crystallography, molecular dynamic simulations and solid-state nuclear magnetic resonance, it selectively responds to the molecular rearrangement of N,N -dimethylformamide, leading to conformation reversion of the flexible ligand, which transfers these actions to deform the whole crystal lattice. These results illustrate that combination of ultramicroporous channel and flexible pore surface could be an effective strategy for the utilization of external physical and chemical stimuli. Porous coordination polymers (PCPs) or metal-organic frameworks have emerged not only as promising adsorbents [1] , [2] , [3] but also as a unique platform for realizing abnormal and controllable physical properties, as they provide remarkable framework flexibility and the host–guest interplay mechanism. For example, a few flexible PCPs showed much larger thermal expansion than common solids because the open coordination frameworks are relatively flexible [4] , [5] , [6] , [7] , [8] , [9] , [10] , [11] , [12] , [13] , [14] , [15] . Whereas small positive thermal expansion (PTE, 0< α <20 × 10 −6 K −1 , α and β V for axial and volumetric thermal expansion coefficients, respectively) is an intrinsic property of common solids [16] , negative (NTE, α <0 K −1 ) [17] , [18] , [19] , [20] , very large (| α |>100 × 10 −6 K −1 ), tunable and other special thermal expansion behaviours are extremely rare and have received considerable theoretical and practical interest [21] , [22] , [23] , [24] , which may be rationally realized by PCPs. However, it is still very challenging to visualize, understand and control the host–guest interplay in porous crystals [15] . The labile nature of guest molecules hinders the precise measurement and control over their locations or motions. Only in exceptional cases, when the host framework retained high crystallinity and the guest molecules were strongly confined, the host–guest interaction could be visualized at the molecular level by X-ray and neutron diffraction techniques [25] , [26] , [27] , [28] , [29] . It is difficult to translate the guest motion to crystal lattice deformation rationally because the thermodynamic energy changes of these two kinds of flexibilities are generally very different in magnitude. To address these issues, we propose a flexible confinement strategy. Ultramicroporous ( Φ <7 Å) [30] channels are well known for their guest confinement and molecular-sieving effects. With suitable pore sizes, they may confine/interact with the adsorbed guest strongly and simultaneously allow the guest motion. A flexible functionality should be decorated on the pore surface to act as a trigger to receive the guest motion and connected with the crystal lattice in a proper way to transfer the local molecular motion to the bulk mechanical response ( Fig. 1 ). Obviously, the key of this strategy is to use a trigger functionality that possesses a potential profile comparable to that of guest motion (that is, thermal energy). 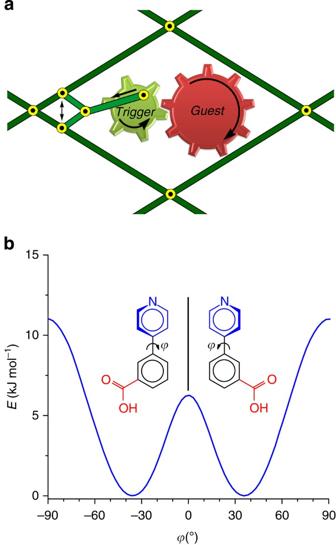Figure 1: Framework and ligand design. (a) The flexible confinement strategy for transforming the guest motion to framework distortion and crystal-shape change. (b) Potential energy profile of Hpba during the pyridyl-ring rotation. Two most stable conformations of the ligand are shown. Figure 1: Framework and ligand design. ( a ) The flexible confinement strategy for transforming the guest motion to framework distortion and crystal-shape change. ( b ) Potential energy profile of Hpba during the pyridyl-ring rotation. Two most stable conformations of the ligand are shown. Full size image Framework construction and analysis We selected 3-(pyridin-4-yl)benzoic acid (Hpba) as a short and flexible ligand for generation of small pores [31] , [32] , [33] , [34] . In a few examples, the biphenyl-like fragments of organic ligands have been observed to undergo paddlewheel movement or conformation change [35] , [36] . The bent backbone of Hpba may transmit/magnify such ligand conformation change to the coordination network via a leverage effect. We calculated the potential energy profile of Hpba at different conformations using the density functional theory ( Fig. 1 ). There are two stable conformations with torsion angles of +35.8 and –35.8° (stereo isomers) between the pyridyl and phenyl rings, which are separated by an energy barrier of 6.3 kJ mol −1 located at the coplanar conformation. The relatively shallow potential wells indicate that the ligand conformation may change easily under external stimuli (such as at different temperatures); however, a conformation reversion should hardly occur below room temperature ( kT =2.5 kJ mol −1 at 300 K) in the absence of more powerful physical (for example, light irritation) or chemical (for example, interaction of other molecules) stimuli [35] , [36] , [37] , [38] . Obviously, such a thermodynamic profile would be suitable for the construction of a temperature–guest-responsive framework. Solvothermal reaction of MnCl 2 and Hpba in N , N -dimethylacetamide (DMA) at 90 °C afforded a metal-carboxylate framework [Mn(pba) 2 ] (MCF-34, 1 ) as colourless needle-shaped crystals. 1 crystallizes in the monoclinic space group I 2/ a , consisting of half of an Mn 2+ ion and one pba − ligand in the asymmetric unit ( Fig. 2 and Supplementary Fig. S1 , Supplementary Table S1 ). Each Mn 2+ ion is coordinated by two N atoms and four O atoms from six pba − ligands, and each pba – is bound to three Mn 2+ ions by an exobidentate carboxylate group and a monodentate pyridyl group, giving a three-dimensional (3D) coordination network with (3,6)-connected ant (anatase) topology. Along the a -axis, Mn 2+ ions are bridged by carboxylate groups to form 1D zigzag Mn-carboxylate chains, which are further bridged by the pyridyl ends of the ligand to form the 3D network, furnishing 1D ultramicroporous channels (void=16.4%, Φ min/max =3.9/4.4 Å) parallel to the Mn-carboxylate chains. 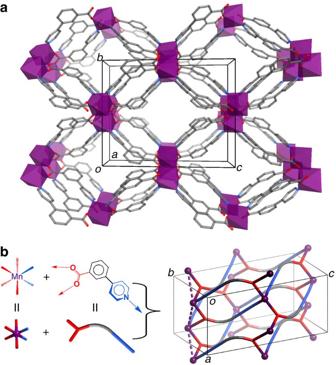Figure 2: Structure of the flexible ultramicroporous coordination framework. (a) X-ray crystal structure of1viewed along its channel direction. (b) Simplification of the coordination framework of1into a (3,6)-connectedantnetwork regarding the tridentate pba–ligand as a three-connected node and the octahedral Mn2+ion as a six-connected node. It can be seen that the fork-like ligand with a bent tail can transfer local structural changes to the distortion of the whole 3D network. For example, breathing of the N−Mn−N angle can change the lengths of theb- andc-axes inversely (not the same magnitude). As the ligand is bent and flexible, its conformation and orientation must change accordingly, which alters the direction of the Mn···Mn vector or the folding degree of the Mn-carboxylate chain (one of which is highlighted by dashed bonds) that determines the length of thea-axis. Figure 2: Structure of the flexible ultramicroporous coordination framework. ( a ) X-ray crystal structure of 1 viewed along its channel direction. ( b ) Simplification of the coordination framework of 1 into a (3,6)-connected ant network regarding the tridentate pba – ligand as a three-connected node and the octahedral Mn 2+ ion as a six-connected node. It can be seen that the fork-like ligand with a bent tail can transfer local structural changes to the distortion of the whole 3D network. For example, breathing of the N−Mn−N angle can change the lengths of the b - and c -axes inversely (not the same magnitude). As the ligand is bent and flexible, its conformation and orientation must change accordingly, which alters the direction of the Mn···Mn vector or the folding degree of the Mn-carboxylate chain (one of which is highlighted by dashed bonds) that determines the length of the a -axis. Full size image Thermogravimetry, infrared spectroscopy and elemental analysis confirmed that 1 was guest-free ( Supplementary Figs S2 and S3 ), indicating that the guest molecules were readily released by routine workup processes. Powder X-ray diffraction (PXRD) showed that 1 can retain framework integrity even after being heated at 673 K for 2 h ( Supplementary Fig. S4 ), which is much higher than those for other organic and organic–inorganic hybrid solids showing large thermal expansion properties [4] , [5] , [6] , [7] , [8] , [9] , [10] , [11] , [12] , [13] , [14] , [15] , [21] , [22] . Gas sorption measurements showed that 1 cannot adsorb N 2 or O 2 at 77 K up to P / P 0 ≈1 but adsorb considerable CO 2 at 195 K, with an apparent Langmuir surface area of 188 m 2 g −1 . However, the CO 2 sorption is very slow, which is also indicated by the hysteric sorption isotherm ( Fig. 3 ). These phenomena may be ascribed to the small channel size and/or large thermal expansion (framework contraction at low temperature). Thermogravimetry and optical microscopy showed that 1 can reversibly adsorb and release many kinds of solvents in the single-crystal to single-crystal manner [39] , [40] . Such highly selective adsorption of solvent/CO 2 over N 2 /O 2 has been observed in a few microporous and ultramicroporous PCPs [41] , [42] , [43] . 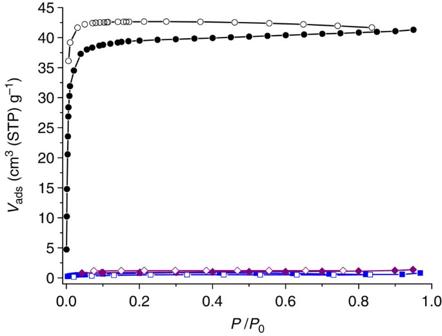Figure 3:Gas adsorption behaviour. N2(blue squares, measured at 77 K), O2(purple diamonds, measured at 77 K) and CO2(black circles, measured at 195 K) adsorption (filled) and desorption (open) isotherms. Figure 3: Gas adsorption behaviour . N 2 (blue squares, measured at 77 K), O 2 (purple diamonds, measured at 77 K) and CO 2 (black circles, measured at 195 K) adsorption (filled) and desorption (open) isotherms. Full size image Thermal expansion properties The thermal expansion behaviours of 1 , both in vacuum and open condition, were studied using single-crystal X-ray diffraction from 127 to 445 K and PXRD from 303 to 673 K ( Supplementary Fig. S5 ). All lattice parameters of 1 change reversibly and linearly against temperature ( Fig. 4 and Supplementary Fig. S6 ; Supplementary Table S2 ). Exceptionally, the b - and c -axes change by +12.0 and –5.3% in a temperature range of about 550 K, corresponding to huge axial PTE and NTE ( α b ′ =+224(1) × 10 −6 K −1 and α c ′ =–107(1) × 10 −6 K −1 , see Table 1 and Supplementary Table S5 ). The thermal expansion profiles obtained for 1 in vacuum and under the open condition were virtually the same, indicating that the thermal expansion property of 1 is not interfered by air adsorption even at low temperatures ( Fig. 3 ). The thermal expansion property of 1 is exceptional because its PTE/NTE coefficients are not only among the largest values for known framework materials [4] , [5] , [6] , [7] , [8] , [9] , [10] , [11] , [12] , [13] , [14] , [15] , [17] but also constant in the widest temperature range even in open conditions. It should be noted that flexible PCPs usually show large (>10%) guest-induced framework breathing [15] , [44] , [45] . When guest occupancy varies with temperature, thermal expansion is overwhelmed by guest-induced framework breathing to produce a nonlinear apparent thermal expansion profile, which is not beneficial for sensor and similar applications [12] , [19] , [20] . This problem is more serious for guest-free PCPs, as they tend to adsorb air (that is, N 2 and O 2 ) especially at low temperatures. For examples, the large isotropic NTE (α =–33.5 × 10 −6 K −1 ) of porous Cd(CN) 2 is constant at 170–375 K, below which it is disturbed by N 2 adsorption [13] . The very flexible PCP FMOF-1 shows the largest linear PTE ( α =+230 × 10 −6 K −1 ) and NTE ( α =–170 × 10 −6 K −1 ) coefficients for framework materials so far but is valid only in vacuum at 90–295 K because it strongly adsorbs N 2 and O 2 (ref. 11 ). 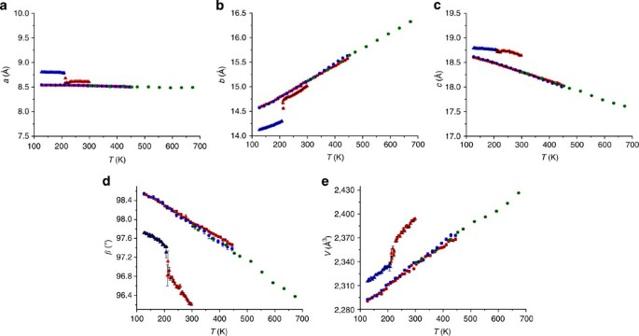Figure 4: Crystal deformation by guest and temperature. (a–e) Temperature-dependent unit-cell parametersa,b,c,βandVfor1-LT·DMF(blue triangle),1-HT·DMF(red triangle),1under N2(blue circle), and1under vacuum (blue circle) measured by single-crystal X-ray diffraction and for1under N2measured by PXRD (green circle). TheaandVvalues of1-LT·DMFare divided by two for comparison with those of other phases. The error bars show the standard deviations. Figure 4: Crystal deformation by guest and temperature. ( a – e ) Temperature-dependent unit-cell parameters a , b , c , β and V for 1-LT·DMF (blue triangle), 1-HT·DMF (red triangle), 1 under N 2 (blue circle), and 1 under vacuum (blue circle) measured by single-crystal X-ray diffraction and for 1 under N 2 measured by PXRD (green circle). The a and V values of 1-LT·DMF are divided by two for comparison with those of other phases. The error bars show the standard deviations. Full size image Table 1 Guest-dependent thermal expansion. Full size table Single-crystal structures of 1 at 127 and 445 K were determined by placing the specimen under cryostat flow without protection ( Supplementary Table S1 ), which further confirmed the high thermal stability and absence of gas adsorption. Comparison of the crystal structures at different temperatures can reveal the structural origins of thermal expansion ( Supplementary Tables S6–S14 ). From 127 to 445 K, the N−Mn−N angle significantly decreases by 4.0°, causing a typical lattice-fence effect to lengthen the b -axis remarkably (the bisector of N−Mn−N angle is parallel to the b -axis) and shorten the c -axis in a smaller magnitude (the N−Mn−N plane has an inclined angle of ca. 39° with the bc -plane). As different parts of the 3D coordination network are interconnected together by the bent ligands, the local structural changes also influence the folding degree of the Mn-carboxylate chains (Mn···Mn separation decreases only 0.013(1) Å, Mn···Mn···Mn angle decreases −0.8°) to slightly increase the length of the a -axis. Guest-responsive crystal lattice deformation The guest-responsive thermal expansion behaviour of 1 was also studied using single-crystal X-ray diffraction. A unique, reversible thermal expansion behaviour was observed for the crystal included with N , N -dimethylformamide ([Mn(pba) 2 ]·0.75DMF or 1·DMF ), which exhibits a phase transition at 208–215 K. In this narrow temperature range, V changes +0.29% meanwhile, and more remarkably, the unit-cell parameters a , b and c change −2.6, +3.0 and −0.20%, respectively [46] , [47] , which in principle could be useful for thermomechanical actuators [22] , [48] . Above the phase transition temperature, 1·DMF adopts the same crystallography symmetry as 1 . Below that, it possesses a lower symmetry ( P 2 1 / c ) with a length-doubled a -axis. For clarity, the high- and low-temperature phases of 1·DMF were denoted as 1-HT·DMF and 1-LT·DMF , respectively ( Fig. 4 and Supplementary Fig. S7 ). The phase-transition temperature (208–215 K) is coincident with the melting point of DMF (212 K), which is quite special considering that confined guests always lose or significantly change their properties of the bulk form (such as the melting point) [49] . The axial and volumetric thermal expansion profiles of 1-LT·DMF below 208 K and 1-HT·DMF above 233 K are linear and similar to those of 1 , indicating that they shared a similar structural mechanism. The thermal expansion magnitude of 1-HT·DMF above 233 K is obviously larger than those of 1 and 1-LT·DMF below 208 K, being consistent with the expectation that the DMF molecules are more mobile at the high-temperature region. Being significantly different from 1 and 1·DMF at other temperatures, all the axes of 1-HT·DMF expand from 215 to 233 K in a fluctuating manner, accompanying a significantly large volumetric thermal expansion ( Supplementary Fig. S7 ). Single-crystal structures of 1·DMF were measured at the representative temperatures of 127, 208, 215, 233 and 294 K ( Supplementary Table S1 and Supplementary Fig. S1 ). The host frameworks of 1-HT·DMF at 215–294 K are isostructural with 1 ; however, 1-LT·DMF at 127–208 K have significant differences with the formers. At the same temperature (294 K), the unit cell slightly expands from 1 to 1-HT·DMF in an anisotropic manner (Δ a / a =+0.8%, Δ b / b =–0.8%, Δ c / c =+1.7%, Δ V / V =+2.1%), accompanying a small increase in the solvent-accessible void from 16.4 to 19.2%. The magnitude of this guest-induced framework breathing is very small among common flexible PCPs [15] , [44] , [45] . In contrast with other examples [11] , [15] , the crystal deformation direction of this guest-induced framework expansion is opposite with that induced by temperature elevation. In this context, the special thermal expansion behaviour of 1-HT·DMF at 215–233 K might be induced by the overwhelming large thermal expansion or relocation of the guest molecules. The guest DMF molecules in crystal structures of 1-HT·DMF are extremely disordered, which could, in principle, arise from thermal motion of the guest molecules and/or symmetry incompatibility between the guest molecules and the host framework. Molecular dynamic simulations showed that there could be many possible DMF locations (with similar energies) at the same pore section in 1-HT·DMF ( Supplementary Fig. S8 ), which is consistent with a statistically (rather than symmetrically) disordered structural model. As indicated by its lower crystal symmetry and larger unit cell, the structural complexity of 1-LT·DMF is four times that of 1 and 1-HT·DMF ( Supplementary Tables S1 and S6–S14 ; Supplementary Fig. S1 ). Two independent DMF molecules can be clearly identified in the crystal structures of 1-LT·DMF , among which, one is completely ordered, whereas another locates at an inversion centre (two-fold disorder, 1/2 occupancy). The symmetry lowering mainly arises from the conformation reversion of one-fourth ligands ( Fig. 5 ). Consequently, the pore surface changes its shape to generate a small pocket, which encloses a methyl group of the completely ordered DMF guest molecule. An abnormal increase in solvent-accessible void was also observed from 1-HT·DMF at 215 K (18.3%) to 1-LT·DMF at 208 K (20.2%), which was related to the generation of additional cavities. Obviously, the pore shape of 1-HT·DMF cannot accommodate a DMF oriented such as in 1-LT·DMF ( Fig. 5 and Supplementary Fig. S9 ). In other words, we have directly observed the thermally induced relocation of guest molecules inside the channel. Similar observations have been only realized in a couple of examples triggered by chemical stimuli such as guest adsorption/desorption [25] , [26] . 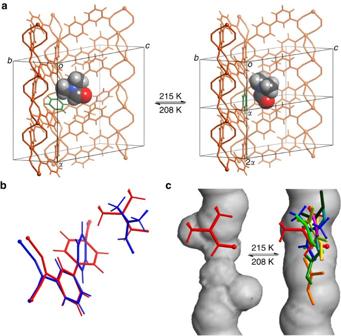Figure 5: Guest relocation induced crystal phase transition. (a) Reversible structure transformation between the LT and HT phases. The pyridyl ring of the ligand showing conformation reversion is highlighted in green, and the related DMF molecule is highlighted in space-filling mode (other DMF molecules are omitted for clarity). (b) Structure alteration of the key local fragments (red: LT phase, blue: HT phase). (c) Change of the pore shape around the conformation-reversing ligand. Several related DMF locations are overlapped above the pore surfaces to compare the host–guest compatibility (red: LT phase, blue: HT phase, other colours without hydrogen atoms: several most possible locations derived from molecular dynamic calculation). Figure 5: Guest relocation induced crystal phase transition. ( a ) Reversible structure transformation between the LT and HT phases. The pyridyl ring of the ligand showing conformation reversion is highlighted in green, and the related DMF molecule is highlighted in space-filling mode (other DMF molecules are omitted for clarity). ( b ) Structure alteration of the key local fragments (red: LT phase, blue: HT phase). ( c ) Change of the pore shape around the conformation-reversing ligand. Several related DMF locations are overlapped above the pore surfaces to compare the host–guest compatibility (red: LT phase, blue: HT phase, other colours without hydrogen atoms: several most possible locations derived from molecular dynamic calculation). Full size image Although the DMF molecules in 1-LT·DMF adopt an ordered arrangement similar to a solid, inside the very narrow 1D channels of 1-HT·DMF , the simple supramolecular chain of DMF molecules should not show identical characteristics of bulk liquids. Nevertheless, the DMF molecules in 1-HT·DMF could still possess much larger and random motion than those in 1-LT·DMF . Variable-temperature solid-state 2 H nuclear magnetic resonance (NMR) measurements were carried out for 1·DMF-d7 (deuterated DMF was used as the guest) to monitor the change of guest motion ( Fig. 6 and Supplementary Figs S10–S12 ). The static 2 H NMR spectra only showed a gradual broadening when the temperature is decreased, which can hardly identify any phase transition. This situation could be probably assigned to the special structure of 1·DMF-d7 , for which the 2 H NMR lineshape depends on not only quadrupolar interaction and dipolar interactions between deuteron and its neighbouring nucleus but also dipolar interaction between deuteron and unpaired electrons. Therefore, we also record the corresponding magic angle spinning (MAS) 2 H NMR spectra. Similar to the static spectra, the envelope of spinning sidebands in the MAS spectra gradually broadens from 294 to 211 K and from 202 to 157 K. However, the width of the envelope decreases dramatically as the temperature is decreased from 211 to 202 K. Meanwhile, the peak width of methyl signal also significantly reduces. These phenomena suggest that DMF molecules adsorbed in 1 might undergo a disorder–order transition as observed in the crystal structures. From 294 to 211 K, the envelope of spinning sidebands in the MAS spectra match well with the static spectra, indicating that the DMF molecules have large thermal motions, which average the chemical shift anisotropy and dipolar interaction even in the static state. From 202 to 157 K, the envelopes of spinning sidebands in the MAS spectra are much narrower than those of the static ones, indicating that the motion of DMF molecules decreased significantly. 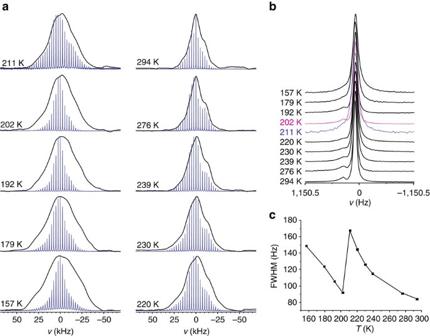Figure 6: Variable-temperature2H NMR spectra. (a) Spectra measured at the static (black, number of scans is 8,000) and MAS (red, spin rate is 2.5 kHz, number of scans is 2,000) modes. (b) Variation of the main peaks of variable-temperature MAS spectra. (c) Evolution of the full width at half maximum (FWHM) of the methyl signal in the MAS spectra. During the HT-to-LT phase transition, the motion of DMF-d7 is significantly slowed down, and a considerable increase in the nucleus–nucleus dipolar interaction and some extent of increase in quadrupolar interaction can be expected, which results in a broadening of the linewidth. On the other hand, the ordering of DMF-d7, as observed in the crystal structures, can narrow the distribution of chemical shifts, which may narrow the linewidth of both static and MAS spectra to some extent. It should be noted that the overall nucleus–nucleus dipolar interaction reflected in the2H NMR spectra stems from a strong dipolar network in a multispin system, although the dipolar interaction is ‘relatively’ weak for each spin pair. Under MAS with a 2.5 kHz sample-spinning rate, the nucleus–nucleus dipolar interaction could be readily suppressed, whereas the quadrupolar interaction and electron–nucleus dipolar interaction (tens of kHz) are only modulated in a smaller extent. Therefore, an obvious narrowing of the envelope of spinning sidebands in the2H MAS spectra is observable when the temperature is decreased from 211 to 202 K. Figure 6: Variable-temperature 2 H NMR spectra. ( a ) Spectra measured at the static (black, number of scans is 8,000) and MAS (red, spin rate is 2.5 kHz, number of scans is 2,000) modes. ( b ) Variation of the main peaks of variable-temperature MAS spectra. ( c ) Evolution of the full width at half maximum (FWHM) of the methyl signal in the MAS spectra. During the HT-to-LT phase transition, the motion of DMF-d7 is significantly slowed down, and a considerable increase in the nucleus–nucleus dipolar interaction and some extent of increase in quadrupolar interaction can be expected, which results in a broadening of the linewidth. On the other hand, the ordering of DMF-d7, as observed in the crystal structures, can narrow the distribution of chemical shifts, which may narrow the linewidth of both static and MAS spectra to some extent. It should be noted that the overall nucleus–nucleus dipolar interaction reflected in the 2 H NMR spectra stems from a strong dipolar network in a multispin system, although the dipolar interaction is ‘relatively’ weak for each spin pair. Under MAS with a 2.5 kHz sample-spinning rate, the nucleus–nucleus dipolar interaction could be readily suppressed, whereas the quadrupolar interaction and electron–nucleus dipolar interaction (tens of kHz) are only modulated in a smaller extent. Therefore, an obvious narrowing of the envelope of spinning sidebands in the 2 H MAS spectra is observable when the temperature is decreased from 211 to 202 K. Full size image The drastic expansion of the b -axis during phase transition is originated from the decrease in the N−Mn−N angle by 1.7°, which is about half that for 1 (4.0°) over a 40 times wider temperature range (320 K). During conformation reversion of the pba – ligand, the large rotation of pyridyl ring actually causes the phenyl ring and sequentially the attached carboxylate group and Mn···Mn vector to rotate in a reversed direction ( Fig. 5 ). These actions significantly increased the folding degree of the Mn-carboxylate chain (Mn···Mn···Mn angle decreased from 128.5 to 122.5°, whereas Mn···Mn separation increased from 4.872 to 4.881 Å), leading to drastic contraction of the a -axis not observed for other instances. Obviously, rotation of the bent ligand also changes its apparent bridging length along the c -axis, which can account for the relatively ‘small’ change of the c -axis. On the other hand, from 215 to 233 K, the structural parameters such as the N−Mn−N angle (+0.15°) and Mn···Mn···Mn angle (+0.1°) change much smaller than the expected values based on the framework-distortion mechanism for 1 and 1·DMF at other temperature ranges, which further exemplifies its special thermal expansion behaviour. Other solvents (DMA, methanol, ethanol, isopropanol and isobutanol) change the crystals’ thermal expansion coefficients in certain extents; however, no phase transition was observed. For example, the volumetric thermal expansion of 1·DMA is slightly larger than 1 , whereas their axial thermal expansion coefficients show more obvious differences ( Table 1 and Supplementary Tables S2–S4 , Supplementary Fig. S13 ). These phenomena indicate that the included guest can generally modulate the thermal expansion magnitude of the host crystal; however, a special crystal phase transition of 1 can be only triggered by DMF selectively. Detailed examination of the crystal structure of 1-LT·DMF showed that the DMF molecule related to the ligand conformation reversion not only embeds one of its methyl groups into the small pocket but also forms multiple weak interactions with other parts of the pore surface and a supramolecular dimer with its symmetry-related neighbour via weak double C−H···O hydrogen bonds between their aldehyde groups ( Supplementary Fig. S14 ). Whereas the molecular sizes and shapes of alcohols (too small or not coplanar) are not suitable for the LT phase pore, the additional methyl group of DMA also prevents the formation of the double C−H···O hydrogen bonds and dimer structure similar to that of DMF. An ultramicroporous framework has been constructed using a conformation-flexible ligand possessing a shallow energy-potential profile. Single-crystal X-ray diffraction studies demonstrated interesting structural responses towards temperature and guest inclusion. Although guest adsorption/desorption alters the host structure very little at room temperature, the thermal expansion properties of the vacant and solvated crystals show great differences. A unique crystal phase transition was observed for the DMF-included crystal, which is related to the conformation reversion of the flexible ligand and is more importantly triggered by the rearrangement of guest molecules. The ultramicroporous structure is crucial for the novel thermal expansion properties, which not only selectively interacts with the DMF molecules strongly to enable the host–guest interplay but also excludes N 2 and O 2 adsorption at low temperatures to extend the effective temperature range for constant and huge thermal expansion of the vacant crystal. This work demonstrated that combination of ultramicropore and framework flexibility could be an effective strategy to design uncommon and controllable thermal-expansion materials. Materials The ligand Hpba was synthesized via the Suzuki–Miyaura coupling reaction with 3-boronobenzoic acid and 4-bromopyridine. Other reagents were commercially available and used without further purification. Measurements Elemental analyses were performed using a Vario EL elemental analyser. Infrared (KBr pellet) spectra were recorded in the range of 400–4,000 cm −1 on a Bruker TENSOR 27 FT-IR spectrometer. Thermogravimetric analyses were carried out using a TA Instruments Q50 analyser under N 2 at a rate of 10 K min −1 . PXRD patterns were recorded with the help of a Bruker D8-Advance diffractometer using Cu Kα radiation and a LynxEye detector. Variable-temperature PXRD analyses were facilitated with an Anton Paar TTK-450 sample stage under N 2 flow (temperature deviation within ca. 2 K). The temperature was increased at a rate of 10 K min −1 and kept for 5 min before measurement at each targeted temperature. Unit-cell parameters were obtained by Pawley refinements using the Reflex module of Materials Studio. Gas sorption isotherms were measured on a Micromeritics ASAP 2020 M physisorption analyser. Ultrahigh-purity-grade (purity >99.999%) N 2 , O 2 and CO 2 gases were used in all adsorption measurements. As-synthesized samples were degassed under high vacuum at 473 K for 3 h before measurement. Temperatures were maintained with liquid nitrogen or dry-ice acetone. Solid-state 2 H NMR spectra were recorded on a Varian Infinityplus-300 spectrometer using a 4-mm double-resonance MAS probe at resonance frequency of 46.0 MHz for 2 H with quadrupolar-echo pulse sequence and a recycle delay of 0.1 s. A typical π /2 pulse length of 2.0 μs was used for 2 H. The sample 1·DMF-d7 was prepared by mixing stoichiometric amounts of guest-free 1 and deuterated DMF (Cambridge Isotope Laboratories, purity 99.5%, containing 0.05% TMS in volume) in a sealed vial. The sample temperatures were calibrated by the chemical shifts of Pb(NO 3 ) 2 (deviation within ca. 5 K), and each spectrum was collected after the targeted temperature had been achieved for 30 min. Synthesis Hpba (0.80 g, 4.0 mmol) was dissolved in DMA (60 ml) using a 250-ml vial, added with a DMA solution of MnCl 2 (0.1 mol l −1 , 20 ml) and methanol (40 ml). The mixture was then sealed with screw cap and heated to 90 °C for 24 h. Colourless needle-like crystals were filtered, washed by methanol and dried in air (yield ca. 80%). Elemental analyses calculated (%) for 1 (C 24 H 15 MnN 2 O 4 ): C 63.87, H 3.57, N 6.21; found: C 63.97, H 3.56, N 6.41. FT-IR (KBr, cm −1 ): 3,420(m), 3,070(w), 2,920(w), 1,660(s), 1,640(s), 1,610(s), 1,500(w), 1,390(s), 1,250(w), 1,220(w), 1,180(w), 1,100(m), 1,040(m), 1,010(m), 839(m), 783(m), 750(m), 708(w), 665(w), 548(m) and 503(m). X-ray single-crystal diffraction Diffraction data were collected on a Bruker APEX CCD diffractometer with graphite-monochromated Mo Kα radiation. To keep constant solvent loading, a single crystal of 1·solvent (just taken out from the solvent) was sealed in a glass capillary. A single crystal of 1 was either sealed in a glass capillary under vacuum or mounted directly on the top of a glass fibre using minimum amount of glue, making sure that most of the crystal surface was exposed to the N 2 flow. The sample temperature was controlled with a dry N 2 open flow using a Rigaku Gas Flow GN2 apparatus (calibrated by a thermal couple at the crystal position, temperature deviation within ca. 2 K). The measurement temperature was changed at 10 K min −1 and kept for 5 min before measurement at each targeted temperature. At each measurement temperature, 3 × 15 diffraction images were collected, and the diffraction spots were indexed to give the unit-cell parameters. Absorption corrections were applied by using the multiscan program SADABS. The crystal structures were solved through the direct method and developed by the difference Fourier technique using the SHELXTL software package. Hydrogen atoms were generated geometrically and refined in a riding model. Anisotropic thermal parameters were applied to all non-hydrogen atoms of the host frameworks in all structures and also to all DMF molecules in 1-LT·DMF at 127 K and one DMF molecule located at the general position in 1-LT·DMF at 208 K. The DMF molecule located at the inversion centre in 1-LT·DMF at 127 K was restrained by a FLAT instruction, whereas that at 208 K was restrained further with several DFIX instructions. DMF/DMA molecules in 1-HT·DMF / 1·DMA were partially located from the difference Fourier maps and manually modelled and restrained in geometry. The occupancies of DMF/DMA molecules in 1·DMF / 1·DMA were refined to be consistent with the results of elementary analyses (Calculated (%) for [Mn(pba) 2 ]·0.75DMF (C 26.25 H 21.25 MnN 2.75 O 4.75 ): C 62.29, H 4.23, N 7.61; found: C 62.25, H 4.28, N 7.27. [Mn(pba) 2 ]·0.75DMA (C 27 H 22.75 MnN 2.75 O 4.75 ): C 62.76, H 4.44, N 7.46; found: C 62.72, H 4.37, N 7.00), thermogravimetry ( Supplementary Fig. S2 ) and molecular dynamic simulations ( Supplementary Figs S8 and S15 ). Calculations Density functional theory calculation was performed at the B3LYP/6-31G(d) level using the Gaussian 03 program. Molecular dynamics was calculated using the Locate task in Sorption module of Materials Studio 5.0 package with Metropolis method based on the universal forcefield. Solvent accessible voids were calculated using the SOLV routine of PLATON. Thermal expansion coefficients of the principal axes ( a ′, b ′ and c ′) were calculated using the PASCal program [50] . Accession codes: The X-ray crystallographic coordinates for structures reported in this Article have been deposited at the Cambridge Crystallographic Data Centre (CCDC) under deposition numbers CCDC 954156-954164. These data can be obtained free of charge from The Cambridge Crystallographic Data Centre via www.ccdc.cam.ac.uk/data_request/cif . How to cite this article: Zhou, H-L. et al . Direct visualization of a guest-triggered crystal deformation based on a flexible ultramicroporous framework. Nat. Commun. 4:2534 doi: 10.1038/ncomms3534 (2013).